Whole-community DNA barcoding reveals a spatio-temporal continuum of biodiversity at species and genetic levels A correlation of species and genetic diversity has been proposed but not uniformly supported. Large-scale DNA barcoding provides qualitatively novel data to test for correlations across hierarchical levels (genes, genealogies and species), and may help to unveil the underlying processes. Here we analyse sequence variation in communities of aquatic beetles across Europe (>5,000 individuals) to test for self-similarity of beta diversity patterns at multiple hierarchical levels. We show that community similarity at all levels decreases exponentially with geographic distance, and initial similarity is correlated with the lineage age, consistent with a molecular clock. Log–log correlations between lineage age, number of lineages, and range sizes, reveal a fractal geometry in time and space, indicating a spatio-temporal continuum of biodiversity across scales. Simulations show that these findings mirror dispersal-constrained models of haplotype distributions. These novel macroecological patterns may be explained by neutral evolutionary processes, acting continuously over time to produce multi-scale regularities of biodiversity. The task of preserving global biodiversity requires both theoretical and empirical understanding of the processes that underpin patterns of species distribution at multiple spatio-temporal scales [1] , [2] , [3] . Biodiversity is a hierarchical concept that embraces multiple levels of biological organization including genes, species and communities [4] . Ideally, models that explain the distribution of diversity should thus invoke processes that apply equally well across various temporal and spatial scales. Early attempts to examine patterns across the biological hierarchy have focused on the link between genetic and species diversity, and have described a correlation between local species richness and intra-specific genetic diversity of species (the species-genetic diversity correlation) [5] . Additional work has extended the species-genetic diversity correlation to other facets of diversity (that is, beta diversity), revealing a correlated distance decay of community similarity on either level [6] . These findings potentially link patterns of biodiversity at different scales via stochastic processes of migration, speciation/mutation and extinction [7] , [8] . An integrated spatio-temporal framework of biodiversity applicable at multiple levels of the biological hierarchy also is emerging from neutral theories of diversity that assume stochastic but spatially limited dispersal as the primary driver of local diversity [9] , [10] . In neutral models, individuals are close to their parents at birth and follow a trajectory of limited dispersal, giving rise to spatial patterns of clumping that may explain macroecological properties at larger scales [11] . Consequently, neutral models have been developed assuming that clumping arises at all spatial scales and hence the distribution of species is self-similar, that is, the proportion of species in an area that are found in a subsection of the area is independent of the area size itself [12] . One of the major challenges to empirical studies across multiple levels of the biological hierarchy is the absence of empirical data. Large-scale DNA sequencing of entire species assemblages provides the means to quantify species and genetic diversity collectively for the members of a given community [6] , [13] , which can be used to test for similarity of patterns across biological levels and broad spatial scales. Here we study genotypic diversity in mitochondrial DNA (mtDNA) in assemblages of aquatic beetles across Europe, spanning c. 30 degrees of latitude. Natural assemblages of aquatic beetles are highly suitable for testing the predictions from dispersal-constrained theoretical models. They form discrete communities of a few dozen species in lakes, ponds and small streams, comprising several families, of which Dytiscidae (predaceous diving beetles) is dominant. Being dependent on open water bodies, dispersal requires discrete migration steps across unsuitable terrestrial habitat. Therefore, using mtDNA sequences for entire local water beetle communities, we investigate if patterns of spatial turnover show self-similarity at multiple hierarchical levels that is predicted under a neutral community ecology paradigm. Our results confirm this expectation, suggesting that a uniform process determines biodiversity patterns across various spatial and temporal scales. Distance decay at species and genetic levels Surveys of 23 regional assemblages ( Fig. 1 , Supplementary Table S1 ) yielded a total of 5,066 sequences and 2,183 unique haplotypes. The Generalized Mixed Yule-Coalescent (GMYC) procedure establishes independently evolving entities [13] that broadly represent the species level [14] . The method grouped total haplotype variation into 274 putative species. The number of species in an assemblage ranged from 13–98 (mean=38, s.d.=20). We first used the species composition of assemblages to test for the decay of assemblage similarity with geographic distance that is expected under a dispersal-constrained model, given continuous dispersion since the origin of lineages [15] . The decline of assemblage similarity with spatial distance was characterized by a simple negative exponential function with halving-distance D 1/2 =1,039 km and initial similarity (intercept with the y-axis) of y =0.64 ( Fig. 1a , Supplementary Table S2 ). We then tested for self-similarity of this pattern at the genotype level, as predicted from a common process that is uniform over time. The haplotype level also showed exponential distance decay but at a much lower initial similarity ( y =0.16) and the decay was slightly faster ( D 1/2 =854 km) than at the species level ( Fig. 1a ). 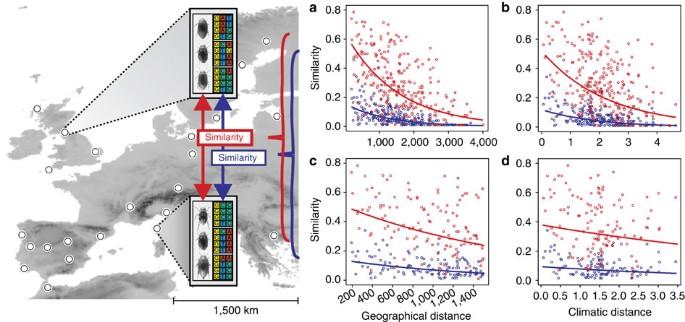Figure 1: Distance decay of similarity in water beetle assemblages across Europe. Fitted curves (species level, red; haplotype level, blue) are exponential decay functions. (a) Decay of similarity against geographic distance across Europe: exponential decay curves were fitted at the species (r2=0.32, Mantel testP<0.001,n=253) and haplotype (r2=0.46,P<0.001) levels. (b) Distance decay of similarity against climatic distance across Europe at the species (r2=0.18,P<0.001,n=253) and haplotype (r2=0.25,P<0.001) levels. (c) Distance decay of similarity against geographic distance for the subset of sites separated by <1,500 km at the species (r2=0.09,P=0.001,n=127) and haplotype (r2=0.13,P=0.001) levels. (d) Distance decay of similarity against climatic distance for the subset of sites separated by <1,500 km at the species (r2=0.02,P=0.07,n=127) and haplotype (r2=0.03,P=0.01) levels. Figure 1: Distance decay of similarity in water beetle assemblages across Europe. Fitted curves (species level, red; haplotype level, blue) are exponential decay functions. ( a ) Decay of similarity against geographic distance across Europe: exponential decay curves were fitted at the species ( r 2 =0.32, Mantel test P <0.001, n =253) and haplotype ( r 2 =0.46, P <0.001) levels. ( b ) Distance decay of similarity against climatic distance across Europe at the species ( r 2 =0.18, P <0.001, n =253) and haplotype ( r 2 =0.25, P <0.001) levels. ( c ) Distance decay of similarity against geographic distance for the subset of sites separated by <1,500 km at the species ( r 2 =0.09, P =0.001, n =127) and haplotype ( r 2 =0.13, P =0.001) levels. ( d ) Distance decay of similarity against climatic distance for the subset of sites separated by <1,500 km at the species ( r 2 =0.02, P =0.07, n =127) and haplotype ( r 2 =0.03, P =0.01) levels. Full size image The decay of similarity at both levels did not stem from the correlation between climatic differences and geographic distance. Given that the steepest decline occurs at shortest geographic distances, we assessed pairs of localities separated by <1,500 km. Over these shorter distances, assemblage similarity was still significantly correlated with geographic distance, but correlation with climatic difference was negligible ( Fig. 1c ). Although other aspects of habitat type or climate not considered here may differ over distances of 1,500 km, our results indicate that the divergence in community composition at this scale can be explained by spatial parameters alone. Distance decay at multiple hierarchical levels We examined the temporal component of self-similarity using the evolutionary information contained in the sequencing data. By reconstructing genealogies within species [16] we can identify the intermediate hierarchical levels between those of species (highest) and haplotypes (lowest). We first established a hierarchical grouping scheme from the mtDNA variation using Templeton’s (1987) algorithm to generate nested clades of n steps according to the number of mutational steps between increasingly more distant haplotypes incorporated into a network [17] . Based on the 2,183 unique haplotypes, the method defined 268 networks, closely matching the number and extent of GMYC groups, as seen elsewhere [18] . Each network contained genealogies of up to five hierarchical levels. The five levels represent a convenient subdivision of lineage history, with the number of groups at each level representing the lineage size at past time intervals. Based on the criteria of the nesting algorithm [17] , the 268 networks (representing the five-step level, hereafter referred to as NC5; Supplementary Table S2 ) were further subdivided into 316, 479, 838 and 1,404 nested groups (NC4, NC3, NC2 and NC1), according to the decreasing number of mutational divergences within each level. When plotting the distance decay of community similarity at each nesting level (as a proxy for clade age), similarity decreased significantly with geographic distance and the shift from one level to the next higher level was largely uniform ( Fig. 2 , see intercepts a in Supplementary Table S2 ). The regularity of the shift between hierarchical levels suggests a uniform underlying evolutionary process. 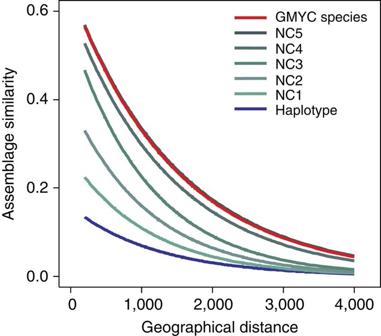Figure 2: Distance decay of similarity of assemblages across Europe at multiple levels. The colour of curves identifies the species (red), haplotype (blue) and intermediate nested-clade (green tones) levels. The fitted lines are exponential decay functions (0.46>r2>0.31, Mantel testP<0.001,n=253). Figure 2: Distance decay of similarity of assemblages across Europe at multiple levels. The colour of curves identifies the species (red), haplotype (blue) and intermediate nested-clade (green tones) levels. The fitted lines are exponential decay functions (0.46> r 2 >0.31, Mantel test P <0.001, n =253). Full size image These analyses of distance decay of similarity were performed with incidence-based methods, but a newly developed index [19] allowed us to assess similarity based on absolute abundance of each entity (from haplotypes to species) among pairs of sites. The abundance-based analysis yielded almost identical results ( Supplementary Fig. S1–S2 ). This finding demonstrates that self-similarity of distance decay at different hierarchical levels also applies to an additional level of complexity concerning species’ abundances in local communities, in addition to incidences of species. From a practical point of view, this suggests that our sampling is a good representation of the studied assemblages because, for abundance data to reveal this pattern, sampling needs to be more detailed to capture the relative proportion of species than to simply record the presence of a species. The fractal geometry of biotic ranges Under neutral dynamics the time since the common ancestor is negatively correlated with the number of lineages, and this correlation is predicted to be linear in a log–log plot indicating fractality [8] . Accordingly, our analysis showed a very strict negative log–log linear correlation ( Fig. 3b ) with slope –1.24. This exponential increment in the number of entities at each hierarchical level is consistent with a fractal pattern. A fractal pattern was also found in the spatial geometry of distribution ranges. The number of entities at each nesting level was tightly correlated with the entities’ range sizes (estimated as the number of occupied sites). Range size showed a very tight correlation with the number of entities at each nesting level in a log–log plot ( Fig. 3c ). Moreover, a striking feature was the great regularity by which the mean similarity and the intercepts of distance decay curves ( Fig. 3d ) declined with the n -step level. This regularity implies that lower-level ranges are uniformly distributed within higher-level ranges throughout the whole phylogenetic history between haplotypes and species. As the n -step level provides an approximate time axis for lineage diversification due to the broadly clock-like rate of change in mtDNA [20] , the correlation with community similarity implies a spatio-temporally continuous process that operates across all hierarchical levels to produce self-similarity at any scale ( Fig. 3a ). These patterns do not simply reflect a constraint of haplotype ranges upon species ranges, as alternative situations are conceivable under which the similarity is higher at lower hierarchical levels ( Supplementary Fig. S3 ). 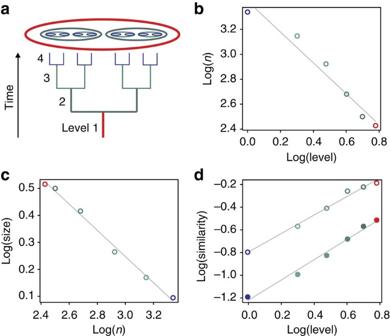Figure 3: Evidence for fractal patterns of biodiversity in time and space. (a) Scheme illustrating how neutral mutations cause a regular branching of lineages through time (molecular clock), and because dispersal is the parameter controlling clade ranges, younger lineages nested in older lineages will have smaller ranges that are regularly nested in older ranges. (b) Observed relationship (linear regressionr2=0.96,F1,4=87.1,P<0.001,n=6) between the number of clades and hierarchical nesting level from haplotypes (level 1) to five-step networks (level 6); (c) Relationship between range size and number of clades (r2=0.99,F1,4=647.4,P<0.001,n=6); (d) Relationship between initial similarity (open circles) and hierarchicaln-step level (r2=0.99,F1,4=364.7,P<0.001,n=6), and between mean similarity (closed circles) and hierarchicaln-step level (r2=0.99,F1,4=407.4,P<0.001,n=6). Red and blue dots represent the species and haplotype levels, respectively, while green tones represent the intermediate nested-clade levels. Grey lines are the fitted functions. Figure 3: Evidence for fractal patterns of biodiversity in time and space. ( a ) Scheme illustrating how neutral mutations cause a regular branching of lineages through time (molecular clock), and because dispersal is the parameter controlling clade ranges, younger lineages nested in older lineages will have smaller ranges that are regularly nested in older ranges. ( b ) Observed relationship (linear regression r 2 =0.96, F 1,4 =87.1, P <0.001, n =6) between the number of clades and hierarchical nesting level from haplotypes (level 1) to five-step networks (level 6); ( c ) Relationship between range size and number of clades ( r 2 =0.99, F 1,4 =647.4, P <0.001, n =6); ( d ) Relationship between initial similarity (open circles) and hierarchical n -step level ( r 2 =0.99, F 1,4 =364.7, P <0.001, n =6), and between mean similarity (closed circles) and hierarchical n -step level ( r 2 =0.99, F 1,4 =407.4, P <0.001, n =6). Red and blue dots represent the species and haplotype levels, respectively, while green tones represent the intermediate nested-clade levels. Grey lines are the fitted functions. Full size image Simulations of neutral against niche-based processes We used simulations to test whether our observed empirical patterns favour dispersal-constrained over niche-constrained scenarios. Communities were simulated that either followed a neutral trajectory of stochastic dispersion and lineage diversification, or that experienced constraints in the dispersion of species by the environment, reflecting niche-constrained conditions (see details in Materials and Methods). The latter disconnects species ranges constrained by niches from the unconstrained dispersion of individuals within the species ranges. Simulated distributions showed that community similarity was correlated with geographic distance at both the species and haplotype levels ( Fig. 4 ), suggesting that migration is at least partially responsible for range size in all cases. Nonetheless, only under neutral conditions were the shapes of the haplotype and species decay curves consistently self-similar; the niche-based model produced increasingly flatter slopes at the haplotype level with reduced community sizes compared with the species level ( Fig. 4 , Supplementary Table S3 ). The correlation of community variation with climatic distance, rather than spatial distance, was weak at both species and haplotype levels ( Supplementary Fig. S4 , Supplementary Table S3 ). Taken together, the dispersal-constrained scenario mirrored the empirical data for European water beetles, whereas the niche-constrained scenario did not. 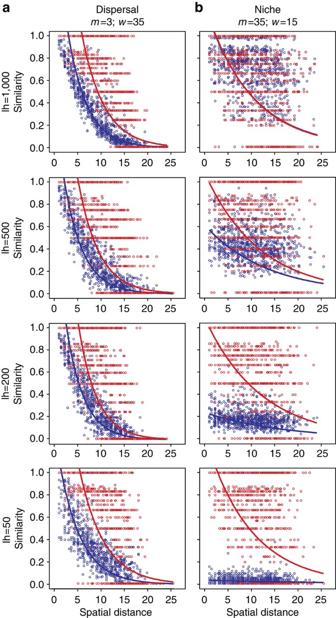Figure 4: Simulations under dispersal- and niche-constrained dynamics. Plots show the decay of similarity with spatial distance for each type of simulation (haplotypes: blue circles and lines; species: red circles and lines) and for different ‘carrying capacities’ in local assemblages (lh). (a) Under the dispersal-constrained scenario, correlation between similarity and spatial distance was always higher than for the niche-constrained scenario. Slopes for the species and haplotype levels were similar for a wide range of carrying capacities when dispersal-constrained, while intercepts were different. (b) Under the niche scenario the slope and intercepts are the same for the species and haplotype levels when the local number of haplotypes is not limited (lh=1,000), while slopes are always flatter for the haplotype level than for the species level when the local number of haplotypes is limited. Figure 4: Simulations under dispersal- and niche-constrained dynamics. Plots show the decay of similarity with spatial distance for each type of simulation (haplotypes: blue circles and lines; species: red circles and lines) and for different ‘carrying capacities’ in local assemblages (lh). ( a ) Under the dispersal-constrained scenario, correlation between similarity and spatial distance was always higher than for the niche-constrained scenario. Slopes for the species and haplotype levels were similar for a wide range of carrying capacities when dispersal-constrained, while intercepts were different. ( b ) Under the niche scenario the slope and intercepts are the same for the species and haplotype levels when the local number of haplotypes is not limited (lh=1,000), while slopes are always flatter for the haplotype level than for the species level when the local number of haplotypes is limited. Full size image The regular shift of the empirical distance decay curves below the species level can be interpreted simultaneously in temporal and spatial dimensions. Spatial distributions of species appear as larger-scale extensions of ranges of lower-level clades (haplotypes and nested clades), while entities at progressively lower nesting levels comprise a set of more recently diversified subordinate lineages. The observed fractal geometry of clade ranges supports the idea that the same neutral processes are underlying the haplotype and species ranges, and the two levels differ in spatial scale only due to the difference in length of time for dispersal (clade age). Existing theoretical models predicting fractal scaling properties of species distributions are based on purely statistical properties [12] , [21] and do not incorporate a mechanistic foundation. Yet, they are consistent with the assumption of stochastic dispersal, birth and death of demographically equivalent individuals of neutral community models [8] that have been shown to produce established species-level macroecological patterns [8] , [9] . The latter models also add a component of neutral evolution, whereby community level abundances determine speciation and extinction probabilities, and, therefore, the longevity of lineages. These differences among lineages determined by metacommunity parameters result in phylogenies that are self-similar at any scale of evolutionary time [8] . Our empirical results not only confirm this pattern of fractal branching in time, but also detect self-similarity in the spatial dimension from the fractal geometry of clade ranges. These findings link the origin of new lineages over time with the spatial structure of lineage ranges across all hierarchical levels, presumably down to the individual. Finally, if the distance decay is explained by individual-based dispersal, this predicts that adjacent communities also are similar in abundance of the member species [8] . This was confirmed here ( Supplementary Fig. S1–S2 ) and further supports the hypothesis of stochastic dispersal. Potentially, non-neutral processes could generate these patterns if environmental factors controlling biotic ranges were spatially structured. There is no evidence for this in the current data, as over a distance of <1,500 km, for which the correlation between spatial distance and climatic difference is very low, environmental differences are negligible to explain the biotic turnover at species and genetic levels ( Supplementary Table S2 ). Our model does not preclude that niche differentiation takes place during the process of dispersal-limited divergence, but it establishes that this is not fundamental to generating the statistical pattern. In addition, haplotype divergences in presumably neutral mtDNA are likely to reflect restricted gene flow among populations in the absence of selection. As the pattern of spatial turnover in these neutral entities is mirrored by the pattern at the species level, this correlation would either be due to complicated dependencies of the (neutral) mtDNA haplotype pattern to follow the (non-neutral) species level pattern, or species-level patterns would also be neutral. As the latter explanation requires only one simple mechanism (stochastic but limited dispersal), the neutral model is a more parsimonious explanation for the reported patterns. The use of neutral markers, such as mtDNA, is a prerequisite for articulating these processes, as the aim was to assess if species ranges, which may be neutral or non-neutral, mirror neutral haplotype ranges. Finally, whereas statistical patterns do not directly inform on the underlying process, we also used simulations to explore mechanistically whether neutral or niche-based processes are able to generate the observed patterns. These simulations suggest that only neutral processes yield the observed patterns, as niche filtering decouples the behaviour of haplotype and species decay curves ( Fig. 4 , Supplementary Fig. S4 ). An integrated spatio-temporal framework of biodiversity can greatly benefit from analyses at the DNA level, linking stochastic population- and species-level processes under common assumptions of migration, speciation/mutation and extinction [5] , [8] . In future, genetic surveys may be supplemented with abundance data to make an explicit link to mechanistic individual-based models of neutral community ecology [22] . A next step will be to assess the generality of the observed patterns in a broad range of taxa. MtDNA haplotype data are generated increasingly for assemblages and entire ecosystems, in particular as part of global DNA barcoding efforts [23] . If evidence for neutrality is obtained generally, this provides a scaffold for biodiversity surveys and comparative analysis. One important consequence of the fractal relationships at multiple levels is that the completeness of sampling at lower genetic levels (for example, total number of haplotypes) can be assessed from regressions through the more completely sampled higher hierarchical groups (see Fig. 3b ). Likewise, the slope of the relationship of range size and hierarchical level ( Fig. 3c ) may be used as a benchmark measure for comparing the spatial scale of community differentiation in various taxa, geographic regions or ecological settings. This slope reflects mean historical dispersal in assemblages, as it measures how neutral ranges expand over time, and hence the rate of past geographical shifts and disturbance of assemblages and ecosystems. Global change of Earth’s biota is increasingly driven by changed dispersal rates due to landscape fragmentation, moving climate zones, metapopulation dynamics after ecosystem disturbance and other factors [24] . A dispersal-based framework of biodiversity that integrates across spatial and temporal scales will reveal global change through its effect on the dispersal dynamics of species assemblages. Sequence data and phylogenetic analysis Each regional assemblage of aquatic beetles along a 4,500-km transect from northern Sweden to Morocco (see Fig. 1 and Supplementary Table S1 ) was composed of several localities within a <50-km radius from both lotic and lentic habitats. Samples were collected in 100% alcohol and identified in the field, to include a total of 204 recognizable species. At every unique locality within a region, all specimens up to a maximum of five individuals per field-identified species were used for DNA extraction. Field identifications were used to maximize the diversity and to obtain a good representation of the total variation, but these identifications were not further utilized. Hence the data reflect the evolutionary history of the target taxa as inferred from a single locus, but any inconsistencies that may result from gene tree–species tree incongruence presumably are avoided due to the very large number of lineages sampled and the relatively rare occurrence of incongruence [25] . Note that with only the mtDNA sequenced, gene tree incongruence could only be assessed indirectly against the morphological species limits; where such incongruence with the mtDNA groups was evident, this usually affected only some portions of the species ranges [26] , that is, any resulting error would affect the details of geographic turnover but not the discovery of species-level groups per se . Genomic DNA was extracted from muscle tissue in the prothorax region with Wizard SV 96-well plates (Promega, UK). An 825 base pair region from the 3′ end of mitochondrial cytochrome oxidase I was amplified with primers Jerry [27] , Ron Inosine, Ron Dyt, Patty, and Pat Dyt [28] . Amplification conditions used with Bioline Taq were 94 °C for 2 min, 35–40 cycles of 94 °C for 30 s, 53 °C for 60 s and 70 °C for 120 s, and a final extension of 70 °C for 10 min. PCR products were cleaned with a 96-well Millipore multiscreen plate, and sequenced in both directions using ABI dye terminator sequencing. Approximately 8,000 individuals were processed. Trace files of forward and reverse strands were analysed with the base calling software Phred [29] under default parameters. Only sequences with >600 bps of Phrap score >20 were retained, resulting in >5,000 high-quality sequences. A small proportion (1.2%) of sequences with indels and in-frame stop codons were removed as putative pseudogenes. A subset of sequences for the subfamily Agabinae was already used in a previous study after manual editing [26] , but the raw data were recompiled here using the automated editing, to make them compatible with all other data. Before tree building, identical haplotypes were collapsed into a single sequence. Gene trees were constructed with RAxML 7.0.3 (ref. 30 ) under the GTR+G+I model selected by jModeltest [31] on a reduced data set (one sequence from one taxonomic species; ∼ 10% of the haplotype-collapsed data set). The maximum likelihood tree was made ultrametric with Pathd8 (ref. 32 ), which implements a mean path length method for establishing a molecular clock. The ultrametric trees were used for quantitative species delimitation with the GMYC method that establishes the point of transition from slow to faster branching rates of the gene tree expected at the species boundary [14] using the R package splits (SPecies LImits by Threshold Statistics) [33] . The GMYC analysis uses the mode of branching to separate intra-specific (coalescent) from inter-specific (Yule) variation [14] and has been widely used to demarcate the species boundary. All genotype information was included in the geographic analysis after application of the GMYC procedure, by restoring (‘uncollapse’) the haplotype data removed before tree building using a custom R script. Minor uncertainty in the haplotype identity due to partially missing sequence data was resolved by randomly assigning the haplotypes to one of the fully sequenced genotypes. Haplotype networks were created from the data set using TCS software [34] implemented in ANeCA v.1.2 (ref. 35 ). TCS uses statistical parsimony to estimate haplotype networks of closely related individuals from DNA sequence data, which is defined by the 95% confidence interval for connections between haplotypes to be non-homoplastic in the network analysis [36] . The nesting algorithm generates n -step hierarchical nested clades of increasingly more inclusive groups of haplotypes, following rules for initially connecting all haplotypes that can be linked by one mutational step (‘1-step networks’), which then are incorporated into groups requiring a connection of maximally two steps (‘2-step networks’), and so on. The procedure implements a stopping rule for the maximum level by which haplotypes are included into a single network based on the probability of encountering homoplastic changes in the connections of two haplotype groups. The large size of the data set required that the TCS software was applied separately to smaller subclades. We, therefore, performed the nested-clade analysis individually on 18 clades defined in a higher-level phylogenetic analysis of Dytiscidae [37] . Custom R and Perl scripts were used for generating relevant input and output files for the various steps. Statistical analysis for empirical patterns Similarity of assemblages among regions (hereafter ‘sites’) was assessed at haplotype, nested clades ( n -step levels) and GMYC (species) levels by means of the Simpson index of similarity, that is, 1-β sim (refs 38 , 39 ), using the R package betapart [40] . To assess the relationship of assemblage similarity with spatial distance and environmental (climatic) differences, nonlinear regression was used to fit exponential decay curves expressed as y = a × e − bx , where y is similarity at distance x , a initial similarity and −b the rate of distance decay. Curves were not forced through the intercept with the y-axis (geographic distance=0). Spatial distance between sites was computed in km as the Euclidian distance between the centroids of regions. Climatic distance was computed as the Euclidian distance in a multidimensional space consisting of three topo-climatic variables, that is, mean altitude, annual mean temperature and annual precipitation [41] that were standardized (mean=0, s.d.=1). These climate variables have proven to be highly correlated to diversity patterns across various taxonomic groups [42] , and were selected here because they yielded the highest correlations with the first three axes in a Principal Coordinate Analysis, that also included other variables as maximum temperature of the warmest month, minimum temperature of the coldest month, precipitation of driest quarter or precipitation of wettest quarter. The degree of association between biotic similarity and spatial or climatic distance was measured as Pearson correlation ( r ) after linearizing the decay curves through log-transformation. An arbitrary small quantity (0.01) was summed to values of similarity=0 to avoid undefined values. Because of possible correlation at large spatial scales, calculations were performed for the full transect, as well as for a reduced data set of pairs of sites separated <1,500 km in which climatic and geographic distance were not closely correlated. The significance of r values was assessed with Mantel tests using the R package vegan [43] . Finally, to assess the robustness of results to variation in abundance, we repeated the aforementioned analyses using a measure of similarity accounting for balanced variation in abundance between localities but independent from abundance gradients: the balanced variation component of Bray–Curtis similarity [19] . This is analogous to Simpson similarity but for abundance data. Simulations of metacommunities Haplotype and species distribution ranges were modelled in a hypothetical landscape to test patterns of species and haplotype composition under alternative processes of stochastic dispersal and niche-based filtering. We were interested in comparing the observed macroecological patterns (which are defined by the presence/absence of clades in a set of localities) against comparable predictions derived from simplified simulations. Given the observed agreement between empirical incidence and abundance-based patterns, there is little gain in simulating the dispersal of individuals, and, therefore, none of the existing individual-based neutral models [22] are applicable here. Instead, we simulated the spread of haplotypes and species ranges with time as a function of migration capacity and the origination of new haplotypes as a function of range sizes. Time and spatial extents of the simulations were arbitrary, but it should be noted that increasing time and spatial extents would be strictly equivalent to reducing the migration parameter. Therefore, our simulations allow exploring the effects of dispersal limitation and niche width in the patterns of haplotype and species turnover. We first defined the landscape by a lattice of 30 × 30 cells, and set two climatic variables (for example, temperature and precipitation), which were partly correlated with spatial dimension x and y by assigning spatial coordinates of 1 to 30 to each cell, and setting values for climate variables to the respective spatial coordinates plus a random value between −10 and 10. This sets the correlation between spatial coordinates and climatic variables to r 2 =0.67. Simulation started with 10 haplotypes, each representing a different species that were located randomly in the landscape. Each haplotype was allowed to disperse according to (i) the dispersal distance m , which was set equal for all haplotypes, and (ii) species niche width w , defined by a maximum distance from the species optimum. Optima were defined as the environmental conditions at the initial, random position of origin of each species. Niche width was a fixed attribute of species that was set equal for all species. Therefore, after origination, the range of the haplotype was allowed to spread to reach all the cells located at spatial distance < m and with climatic conditions differing from the optimum < w . We repeated the simulation for three different dispersal capacities ( m =3, 5, 35) combined with three different niche widths ( w =10, 15, 35). A further parameter was set to control the size of local assemblages. Given that abundances were not modelled, we set a limit to the number of local haplotypes (lhs) as a surrogate. Simulations were replicated for lh values between 50 and 1,000 lhs, representing highly saturated to completely unsaturated local assemblages. Origination of new lineages was simulated at a given time by adding new haplotypes at random points within the existing species ranges, with the mutation rate constant per cell occupied. New and old haplotypes continued to disperse as defined by m . This process of sequential origin of new haplotypes and subsequent expansion of their ranges was repeated until each species included haplotypes of four different ages (hierarchical levels) and, consequently, four different range sizes. To avoid edge effects, we did not score the outer five rows of cells at each side of the lattice, so subsequent analyses were performed within the central 20 × 20 cells ( n =400). Again, it should be noted that allowing more origination/spread cycles would be strictly equivalent to increasing the migration parameter, which was allowed to vary from strong dispersal limitation to unlimited dispersal to cope with all situations. We then computed Simpson similarity between all pairs of cells at the species and haplotype levels, fitted exponential decay curves to test the variation explained ( r 2 ) by spatial and climatic distance, and assessed its significance with a Mantel test (see above). Note that a low dispersal rate combined with a wide niche is equivalent to a dispersal-constrained model, whereas under high dispersal combined with narrow niche width species ranges are controlled almost exclusively by climate. All simulations were performed in R [44] . Accession codes: Sequences have been deposited in EMBL Protein Knowledgebase database under accession numbers JN840019 - JN845080 . How to cite this article: Baselga, A. et al. Whole-community DNA barcoding reveals a spatio-temporal continuum of biodiversity at species and genetic levels. Nat. Commun. 4:1892 doi: 10.1038/ncomms2881 (2013).